Probing dark exciton diffusion using photovoltage The migration of weakly and non-luminescent (dark) excitons remains an understudied subset of exciton dynamics in molecular thin films. Inaccessible via photoluminescence, these states are often probed using photocurrent methods that require efficient charge collection. Here we probe exciton harvesting in both luminescent and dark materials using a photovoltage-based technique. Transient photovoltage permits a real-time measurement of the number of charges in an organic photovoltaic cell, while avoiding non-geminate recombination losses. The extracted exciton diffusion lengths are found to be similar to those determined using photocurrent. For the luminescent material boron subphthalocyanine chloride, the photovoltage determined diffusion length is less than that extracted from photoluminescence. This indicates that while photovoltage circumvents non-geminate losses, geminate recombination at the donor–acceptor interface remains the primary recombination pathway. Photovoltage thus offers a general approach for extracting a device-relevant diffusion length, while also providing insight in to the dominant carrier recombination pathways. As a quasi-particle with no net charge, excitons are difficult to probe directly by electrical means. This is particularly true in organic semiconductors where the exciton binding energy is ∼ 1 electronvolt [1] , [2] . As such, devices constructed using these materials are often intrinsically excitonic, and the properties of the exciton strongly determine device design and functionality [3] , [4] , [5] , [6] , [7] , [8] , [9] . Consequently, knowledge of exciton behaviour is essential in order to properly interpret material and device physics. This has been especially true in the evolution of organic photovoltaic cell (OPV) design. In an OPV, excitons must diffuse from the point of photogeneration to an electron donor–acceptor (D–A) interface in order to be dissociated and collected as a photocurrent [1] , [2] , [10] . Indeed, much effort has been directed at characterizing exciton transport and measuring the characteristic exciton diffusion length ( L D ). Such measurements often rely on tracking the end-of-life products of the exciton, namely, photons or charge carriers [11] , [12] , [13] , [14] , [15] , [16] , [17] , [18] , [19] . In steady-state photoluminescence (PL)-based measurements of L D , emitted photons represent excitons that fail to reach the dissociating interface. The ratio of steady-state PL from a film with a dissociating interface to the PL from a film without a dissociating interface is equivalent to the ratio of exciton densities in the two films, and can be modelled using a diffusion equation to extract L D [3] , [11] , [12] , [20] , [21] , [22] . Measurements of transient PL can also reveal similar insights into exciton transport, based on a reduction in the exciton lifetime due to interaction with a quencher [16] , [23] , [24] . Despite the popularity of PL-based measurements of exciton transport, they are incapable of probing the dynamics of singlet or triplet excitons with exceedingly low luminescence quantum yields. Charge carrier based techniques are capable of probing materials with low luminescence efficiencies, however these measurements can require involved experimental techniques, non-device relevant architectures or are subject to charge collection losses [2] , [18] , [19] , [20] , [25] . The most straightforward of these approaches are photocurrent-based measurements, where device external quantum efficiency ( η EQE ) spectra are fit for L D by combining rigorous simulations of the generating optical field with a diffusion equation [2] , [20] , [25] . While excellent fits to the experimental data can be realized, losses due to geminate recombination at the D–A interface as well as non-geminate recombination during the charge collection process are often ignored [2] , [20] , [26] . This approximation can result in underestimates in the extracted value of L D whenever the overall charge collection efficiency ( η CC ) <1. Fitting of η EQE spectra is thus only expected to yield a value of L D comparable to PL measurements in the absence of all recombination losses. Instead of extracting carriers as photocurrent, we measure the number of carriers immediately after generation using photovoltage. Exciton dissociation leads to the initial formation of a charge transfer state at the D–A interface, followed by dissociation of the charge transfer state into mobile carriers. Indeed, dissociation of the charge transfer state may compete with rapid geminate recombination at the interface. Once dissociated, charge carriers occupy sites of disparate potential energy, leading to the generation of a measurable voltage. The magnitude of the voltage generated by an OPV is proportional to the number of charge carriers in the donor and acceptor active layers [27] , [28] , [29] . To measure L D using a photovoltage-based technique, the exact relationship between the number of charge carriers and voltage must be known, and it must also be demonstrated that non-geminate recombination losses are negligible. Since charge transfer states that undergo rapid recombination will not accumulate in numbers sufficient to generate a measureable photovoltage, losses related to geminate recombination are included in the photovoltage measurement. Here the L D of boron subphthalocyanine chloride (SubPc, Fig. 1a ) and C 60 are measured using photovoltage, and the value for SubPc is compared with previous PL-based measurements. The technique is then employed to measure L D for several dark phthalocyanine materials, which are inaccessible using PL methods. 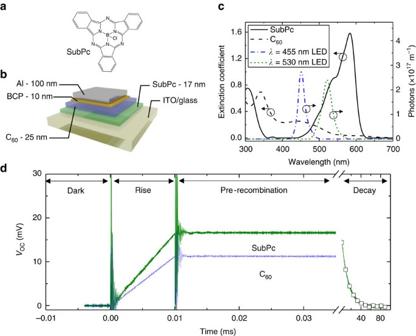Figure 1: Photovoltage response for a SubPc-C60planar heterojunction OPV. (a) Molecular structure of SubPc and (b) architecture for the SubPc-C60OPV. (c) Pump spectra for LEDs peaked at wavelengths ofλ=455 nm andλ=530 nm compared with the thin film extinction coefficients of SubPc and C60. (d) Representative plot of the open-circuit voltage response to a 10 μs incident light pulse showing four data sets. There are two data sets shown in the regions labelled Dark, Rise and Pre-recombination, where SubPc data is shown in green and C60data is shown in blue. The region labelled ‘Decay’ shows two photovoltage decays, one is for primarily pumping C60(squares) and one for primarily pumping SubPc (green line in decay). Both decays correspond to a peak voltage of 16.5 mV and have time constants of∼14 ms. The equivalence of the decays demonstrates that the photovoltage decay only depends on the number of carriers and not which material is being pumped. Figure 1: Photovoltage response for a SubPc-C 60 planar heterojunction OPV. ( a ) Molecular structure of SubPc and ( b ) architecture for the SubPc-C 60 OPV. ( c ) Pump spectra for LEDs peaked at wavelengths of λ =455 nm and λ =530 nm compared with the thin film extinction coefficients of SubPc and C 60 . ( d ) Representative plot of the open-circuit voltage response to a 10 μs incident light pulse showing four data sets. There are two data sets shown in the regions labelled Dark, Rise and Pre-recombination, where SubPc data is shown in green and C 60 data is shown in blue. The region labelled ‘Decay’ shows two photovoltage decays, one is for primarily pumping C 60 (squares) and one for primarily pumping SubPc (green line in decay). Both decays correspond to a peak voltage of 16.5 mV and have time constants of ∼ 14 ms. The equivalence of the decays demonstrates that the photovoltage decay only depends on the number of carriers and not which material is being pumped. Full size image Probing exciton diffusion with photovoltage Figure 1b shows the device architecture used to demonstrate the photovoltage-based technique for measuring L D . The OPV is a planar heterojunction device comprised of the electron donating material SubPc paired with the electron accepting material C 60 . The device is capped with an exciton blocking layer of bathocuproine (BCP) and a 100-nm-thick aluminum (Al) cathode. While the focus of this work lies in applying the photovoltage-based technique to dark materials, SubPc serves as a useful starting point since L D has been previously measured by PL-based techniques [3] , [12] . For the device of Fig. 1b , SubPc or C 60 can be probed by varying the pump light-emitting diode (LED) spectrum. The extinction coefficients of SubPc and C 60 are shown in Fig. 1c , along with the emission spectra of two LEDs: a blue LED ( λ peak =455 nm) used to primarily excite C 60 and a green LED ( λ peak =530 nm) used to excite SubPc. When the SubPc-C 60 device is held at open-circuit and excited by one of the LEDs for 10 μs, the resulting photovoltage response is shown in Fig. 1d . Since SubPc and C 60 do not have completely distinct extinction coefficients, excitons originating on SubPc comprise about 79% and 9% of the photovoltage response for the green and blue LED pulses, respectively [20] . The photovoltage response of Fig. 1d is characterized by four regions termed dark, rise, pre-recombination, and decay. In the dark region, the LED is off and there are no carriers present in the device, corresponding to zero photovoltage. During the rise phase, the LED is on, leading to exciton generation in the OPV, some of which undergo charge transfer at the D–A interface to generate charge carriers. The accumulation of charge carriers generates the linear voltage rise. Once generated, there is a rate for charge carriers to undergo recombination, leading to the photovoltage decrease shown in the decay region. The eventual decay in photovoltage is attributed to non-geminate charge carrier recombination, and is slow enough that a measure of the photovoltage can be made before any substantial number of charge carriers recombine. This is demonstrated by the photovoltage ‘plateau’ observed at short times in the pre-recombination region of Fig. 1d . The behaviour in Fig. 1d can be approximated by different regimes of the rate equation governing the number of carriers ( n ) in the OPV: In equation (1), G is the generation rate of charge carriers, τ rec is the non-geminate, charge carrier recombination time, and α represents the order of recombination [30] . The terms on the right of equation (1), refer to the corresponding regions of Fig. 1d . The plateau observed in Fig. 1d verifies that τ rec is sufficiently long such that no significant charge carrier recombination occurs during the LED pulse. In other words, the plateau persists for a time longer than the LED pulse time. As long as the voltage is measured before the plateau begins to decay, only negligible recombination has occurred which enables an accurate measure of the number of charge carriers generated at the interface. Relating photovoltage to the number of charge carriers In order to extract a diffusion length from photovoltage data, the curves of Fig. 1d must be translated into a measurement of the number of charge carriers present in the device. The relationship between photovoltage and the number of charge carriers is non-trivial to calculate [27] , [28] , but it can be directly measured using charge extraction methods [31] , [32] , [33] . While the charge extraction approach is employed here, any means of relating the number of charge carriers to the device voltage could be used instead of charge extraction. In a charge extraction experiment, the OPV is illuminated and held at open-circuit. Once the steady-state voltage is reached and recorded, the OPV is switched to short-circuit and the resulting current transient is recorded. The integral of the current transient yields the number of charge carriers extracted from the cell as well as the relationship between the number of carriers and the photovoltage [29] , [34] . 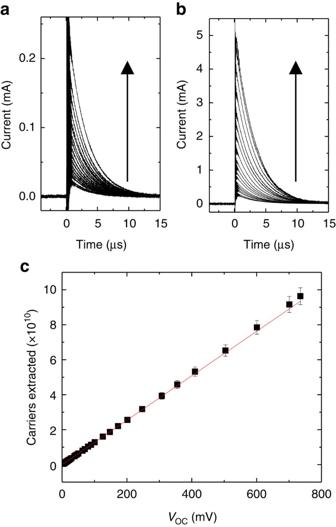Figure 2: Charge extraction to relate photovoltage and number of charge carriers. (a,b) Current transients obtained by switching the SubPc-C60device inFig. 1bfrom open-circuit (steady-state) to short-circuit. The arrow points in the direction of increasing optical illumination and hence,VOCbefore switching to short-circuit. In (a), theVOCis varied from 3.4 mV to 37.6 mV while in (b), theVOCis varied from 40.8 mV to 735 mV. (c) The trend of carrier number as a function of photovoltage obtained by integrating parts (a) and (b) with respect to time. A linear fit (solid red line) to the data is also shown with an intercept of zero and a slope of 1.27 × 1011carriers per Volt. The error bars represent the standard deviation across eight devices. Figure 2a,b show current transients, recorded for the SubPc-C 60 device of Fig. 1b , as a function of illumination intensity. As the illumination is increased (leading to a larger V OC ), the total current extracted from the device increases. Figure 2a shows the current transients for V OC values ranging from 3.4 to 37.6 mV while Fig. 2b shows higher V OC values from 40.8 to 735 mV (peak V OC values for each scan in Fig. 2 are listed in the Supplementary Note 1 ). Fig. 2c shows the current transients integrated with respect to time yielding the number of charges stored in the device for a given photovoltage. Due to the fast extraction of carriers in the charge extraction experiment, Fig. 2c is the measured number of carriers in the OPV as a function of V OC (ref. 31 ). Thus, with this plot, any measure of photovoltage can be translated into a measure of the number of charge carriers present in the device. While it may be assumed that some charges will undergo recombination before being extracted during the charge extraction measurement, the characteristic extraction time of about 5 μs is significantly shorter than the characteristic recombination time shown in Fig. 1d . Thus, we conclude that the impact of charge carrier recombination on the charge extraction measurement is negligible, in agreement with a previous analysis [31] . Figure 2: Charge extraction to relate photovoltage and number of charge carriers. ( a , b ) Current transients obtained by switching the SubPc-C 60 device in Fig. 1b from open-circuit (steady-state) to short-circuit. The arrow points in the direction of increasing optical illumination and hence, V OC before switching to short-circuit. In ( a ), the V OC is varied from 3.4 mV to 37.6 mV while in ( b ), the V OC is varied from 40.8 mV to 735 mV. ( c ) The trend of carrier number as a function of photovoltage obtained by integrating parts ( a ) and ( b ) with respect to time. A linear fit (solid red line) to the data is also shown with an intercept of zero and a slope of 1.27 × 10 11 carriers per Volt. The error bars represent the standard deviation across eight devices. Full size image Extracting the exciton diffusion length With an experimental relationship between the photovoltage and the number of carriers ( Fig. 2c ), as well as the knowledge that recombination can be ignored, L D can be determined for SubPc from the transient photovoltage data of Fig. 1d . The optical pump pulse spectrum is measured with a spectrometer, and the pulse power is measured using a silicon photodiode to determine that the green ( λ peak =530 nm) pulse in Fig. 3a contains 8.64 × 10 9 photons. Some of the excitons generated from the pulse reach the interface and dissociate into charge carriers, leading to the observed voltage rise in Fig. 1d . The data in Fig. 2c can then be referenced to determine that 2.09 × 10 9 carriers are generated for the observed voltage plateau of 16.6 mV. Since non-geminate recombination is negligible, this also means that 2.09 × 10 9 excitons were dissociated into separated charge carriers. 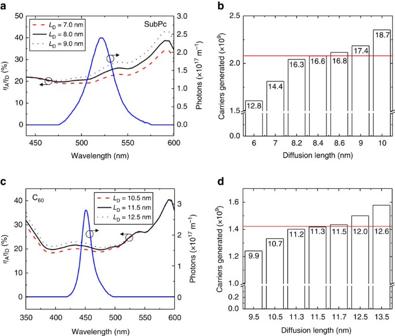Figure 3: ExtractingLDfrom the number of carriers measured by photovoltage. (a) SimulatedηAηDfor variable values of the SubPcLD, with a constant C60LDof 11.5 nm. Also shown, is the total number of photons incident on the device over a 10 μs pulse (solid blue line). (b) The number of charge carriers predicted to be generated for different SubPcLDvalues. The horizontal line (red) marks the experimentally measured number of charge carriers generated. The labels on the bars represent the photovoltage (in millivolts) the device would generate for each value ofLD,showing the sensitivity of the technique. (c) SimulatedηAηDfor variable values of the C60LD, with a constant SubPcLDof 8.4 nm, and the total number of incident photons over a 10 μs pulse (solid blue line). (d) The predicted number of generated charge carriers for different values of the C60LD. The horizontal line (red) marks the experimentally measured number of charge carriers generated, while the bar labels represent the generated photovoltage (in millivolts) for each value ofLD. Figure 3: Extracting L D from the number of carriers measured by photovoltage. ( a ) Simulated η A η D for variable values of the SubPc L D , with a constant C 60 L D of 11.5 nm. Also shown, is the total number of photons incident on the device over a 10 μs pulse (solid blue line). ( b ) The number of charge carriers predicted to be generated for different SubPc L D values. The horizontal line (red) marks the experimentally measured number of charge carriers generated. The labels on the bars represent the photovoltage (in millivolts) the device would generate for each value of L D, showing the sensitivity of the technique. ( c ) Simulated η A η D for variable values of the C 60 L D , with a constant SubPc L D of 8.4 nm, and the total number of incident photons over a 10 μs pulse (solid blue line). ( d ) The predicted number of generated charge carriers for different values of the C 60 L D . The horizontal line (red) marks the experimentally measured number of charge carriers generated, while the bar labels represent the generated photovoltage (in millivolts) for each value of L D . Full size image To extract L D from the measured number of dissociated excitons, the absorption efficiency ( η A ) and the diffusion efficiency ( η D ) must also be known. A transfer matrix formalism is used to calculate η A and the exciton generation profile as a function of incident photon wavelength ( λ ) (ref. 20 ). From the generation profile, the exciton diffusion equation can be used to calculate η D ( λ , L D ). Example calculations of η A η D are shown in Fig. 3a for varying values of the SubPc L D . Multiplying η A η D by the number of incident photons ( P inc ) and integrating yields the number of carriers that would be generated by exciton dissociation ( n gen ) as a function of L D : Figure 3b is obtained by applying equation (2) to simulated η A η D traces like the ones shown in Fig. 3a . When the correct value of L D is used, the integral of equation (2) matches the measured number of excitons dissociated (2.09 × 10 9 as determined from the photovoltage transient), and the diffusion length is determined. In this example, the L D of SubPc is determined to be 8.4 nm. The same analysis can be performed for C 60 using the C 60 voltage transient of Fig. 1d . The LED pump spectrum is shown in Fig. 3c along with a series of simulated η A η D curves. When equation (2) is applied to the curves in Fig. 3c, Fig. 3d is generated. In this example, the diffusion length of C 60 is found to be 11.5 nm for the V OC transient of Fig. 1d . Figure 3b,d demonstrate the sensitivity of the photovoltage-based approach. Each bar is labelled by the photovoltage (in mV) that would be measured for the corresponding L D and number of charge carriers generated. The oscilloscope employed here to measure voltage has a resolution of ∼ 0.2 mV which gives an L D resolution of about±0.2 nm for the device in Fig. 1b . While the diffusion length can be determined within this small error for a given device, there remain uncontrolled effects in device fabrication that lead to more substantial device-to-device deviations. As such, the standard deviation is taken as the error in L D . By averaging across twelve devices, L D values of (8.5±1.0) nm and (11.5±1.2) nm are obtained for SubPc and C 60 , respectively. Active layer thicknesses for all devices considered in this study are included in the Supplementary Note 2 . To put these values into context, the η EQE was also measured for the SubPc-C 60 device of Fig. 1b and is shown in Fig. 4 . When this η EQE data is compared with a prediction using an optical transfer matrix formalism and exciton diffusion equation with the photovoltage determined values of L D [20] , excellent agreement is observed. Direct fitting of the η EQE data using the same model yields L D values of 8.0 and 12.2 nm for SubPc and C 60 , respectively, similar to those obtained from photovoltage. This agreement occurs despite the fact that the measurement of η EQE may include non-geminate recombination losses, which are circumvented in the photovoltage measurement. These results suggest that non-geminate recombination losses are negligible in planar heterojunction OPVs based on SubPc-C 60 near short-circuit. Thus, the charge collection efficiency at short-circuit is dominated by geminate recombination losses [34] . 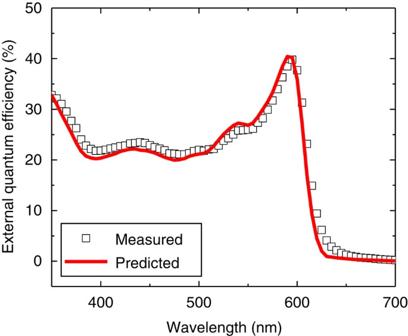Figure 4: Comparing photovoltage-determined values ofLDtoηEQE. Comparison of the measured deviceηEQEto that predicted usingLDvalues extracted from photovoltage withηCC=1. Since the measurement ofLDintrinsically reflects the impact of geminate recombination, the agreement between the measured and simulatedηEQEsuggests that non-geminate recombination is negligible in this device at short circuit. Figure 4: Comparing photovoltage-determined values of L D to η EQE . Comparison of the measured device η EQE to that predicted using L D values extracted from photovoltage with η CC =1. Since the measurement of L D intrinsically reflects the impact of geminate recombination, the agreement between the measured and simulated η EQE suggests that non-geminate recombination is negligible in this device at short circuit. Full size image It is instructive to compare the photovoltage-extracted L D for SubPc to that obtained from conventional thickness-dependent PL quenching. PL quenching involves the tracking of PL as a measure of excitons that do not reach the D–A interface. This measurement is subtly different than the photovoltage approach in that the photovoltage is only sensitive to excitons that reach the interface, dissociate, and yield charge carriers that contribute to the voltage. Indeed, while excitons that form charge transfer states and undergo rapid geminate recombination will not contribute substantially to the photovoltage, these states will contribute to a reduction in PL. As such, materials and architectures that exhibit rapid geminate recombination should yield a different value of L D depending on the method applied. Previous reports for SubPc place its diffusion length in the range of L D =10.7 nm, larger than the results reported here using photovoltage [3] . As noted, this disagreement suggests that there is substantial geminate recombination present at the D–A interface, and that the value extracted from photovoltage is as a result, an underestimate to the intrinsic L D of SubPc. It is worth noting that in materials with substantial exciton-exciton or exciton-polaron quenching, these losses will also be reflected in L D . Here no variation in L D is observed with active layer thickness or light intensity [35] . In cases where geminate recombination plagues a planar heterojunction device of interest, the extracted L D still represents the extractable fraction of excitons dissociating at the D–A heterojunction. Measuring dark exciton transport in phthalocyanine devices While the discussion hereto has focused on the luminescent donor material SubPc to demonstrate the photovoltage technique, the method is broadly applicable provided the material of interest can be used as either a donor or acceptor layer in a planar heterojunction OPV ( id est , it produces a photovoltage) without need to optimize the device or reach high efficiency. As demonstrated with C 60 , the photovoltage technique is capable of probing the L D of dark excitons. Here, we further demonstrate this by extracting the L D of the archetypal donor material copper phthalocyanine (CuPc). 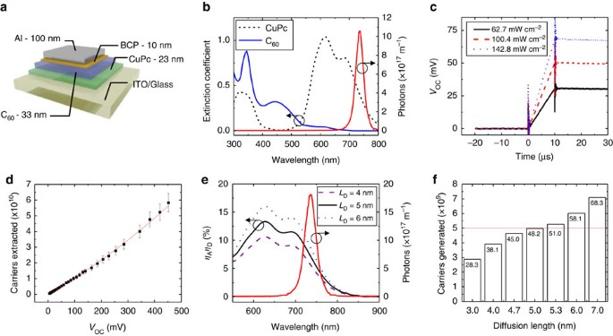Figure 5: Measuring theLDof CuPc. (a) Architecture for the planar heterojunction OPV based on the donor-acceptor pairing of CuPc-C60. (b) Comparison of the extinction coefficients for CuPc and C60as well as the spectrum of the LED pulse (λpeak=735 nm) used to pump CuPc. (c) Photovoltage rises recorded when pumping CuPc with theλ=735 nm LED at intensities of 62.7 mW cm−2(black), 100.4 mW cm−2(red) and 142.8 mW cm−2(blue). (d) Relationship between charge carriers and voltage in the CuPc-C60device obtained using the charge extraction method and an exponential fit to the data. The error bars represent the standard deviation across eight devices. (e) SimulatedηAηDcurves for three CuPcLDvalues with a constant C60LDof 12.1 nm compared with the time integrated LED pump spectrum. (f) Comparison of the predicted number of charge carriers generated (for multiple values of the CuPcLD) to the photovoltage-based measurement (horizontal line). TheVOC(in millivolts) that would be measured for the corresponding number of charge carriers is labelled for each bar. Figure 5a shows the device structure used, consisting of a heterojunction between CuPc and C 60 , and Fig. 5b demonstrates that nearly all of the pump LED ( λ peak =735 nm) is absorbed by CuPc. Three voltage transients for 10 μs pulses of varying intensity are shown in Fig. 5c . As the intensity of the LED pulse increases, the photovoltage response of the device plateaus at larger voltages. Using Fig. 5d this can be related to an increased number of charge carriers being generated at the D–A interface. As demonstrated for SubPc and C 60 , the L D can be extracted using Fig. 5c,d . Figure 5e shows the calculated η A η D for three possible L D values overlaid with the LED spectrum at an intensity of 100.4 mW cm −2 . Figure 5f gives the results of applying equation (2) to a series of these η A η D curves for the pump shown in Fig. 5e . In this example, a diffusion length of 5.0 nm is extracted for CuPc. This value agrees well with the L D extracted for the other pump intensities shown in Fig. 5c : L D =4.94 nm for 62.7 mW cm −2 and L D =4.97 nm for 142.8 mW cm −2 . Figure 5: Measuring the L D of CuPc. ( a ) Architecture for the planar heterojunction OPV based on the donor-acceptor pairing of CuPc-C 60 . ( b ) Comparison of the extinction coefficients for CuPc and C 60 as well as the spectrum of the LED pulse ( λ peak =735 nm) used to pump CuPc. ( c ) Photovoltage rises recorded when pumping CuPc with the λ =735 nm LED at intensities of 62.7 mW cm −2 (black), 100.4 mW cm −2 (red) and 142.8 mW cm −2 (blue). ( d ) Relationship between charge carriers and voltage in the CuPc-C 60 device obtained using the charge extraction method and an exponential fit to the data. The error bars represent the standard deviation across eight devices. ( e ) Simulated η A η D curves for three CuPc L D values with a constant C 60 L D of 12.1 nm compared with the time integrated LED pump spectrum. ( f ) Comparison of the predicted number of charge carriers generated (for multiple values of the CuPc L D ) to the photovoltage-based measurement (horizontal line). The V OC (in millivolts) that would be measured for the corresponding number of charge carriers is labelled for each bar. 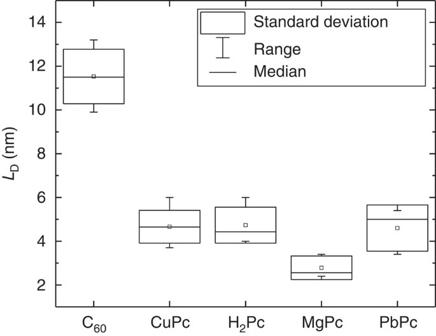Figure 6: Comparison ofLDvalues obtained using photovoltage. Values ofLDextracted using the photovoltage-based technique for C60and a series of phthalocyanine molecules differing in the coordinating metal atom: metal-free (H2Pc), magnesium (MgPc), copper (CuPc) and lead (PbPc). The small square symbol represents the mean of all measured devices and the boxes represent the standard deviation across all measured devices. Full size image Figure 6 shows the L D extracted for a variety of dark materials using photovoltage. In addition to C 60 , a series of phthalocyanine molecules differing only in the central coordinating metal atom are shown: metal-free (H 2 Pc) L D =4.7 nm ( Supplementary Fig. 1 ), magnesium (MgPc) L D =2.8 nm ( Supplementary Fig. 2 ), copper (CuPc) L D =4.7 nm, and lead (PbPc) L D =4.6 nm ( Supplementary Fig. 3 ). Besides demonstrating the wide applicability of the photovoltage-based L D technique, Fig. 6 demonstrates an interesting trend. The average L D of all of the phthalocyanine molecules fall within a range of about two nanometers despite the nature of the exciton in these molecules differing as a function of the coordinating metal atom. The exciton in H 2 Pc is likely a singlet exciton with a lifetime of about 250 ps, whereas the excitons in CuPc and PbPc are likely long-lived triplet excitons [24] . The sharing of a crystal structure between H 2 Pc and CuPc further makes the similar exciton diffusion length of interest as these two materials provide a unique opportunity to contrast the motion of singlet and triplet excitons in very similar environments. Figure 6: Comparison of L D values obtained using photovoltage. Values of L D extracted using the photovoltage-based technique for C 60 and a series of phthalocyanine molecules differing in the coordinating metal atom: metal-free (H 2 Pc), magnesium (MgPc), copper (CuPc) and lead (PbPc). The small square symbol represents the mean of all measured devices and the boxes represent the standard deviation across all measured devices. Full size image This work demonstrates an alternate, photovoltage-based method for probing exciton harvesting that is applicable to any material that can facilitate exciton dissociation at the heterojunction in a planar OPV. The approach utilizes a unique understanding of the information contained in the photovoltage of an OPV to measure the number of charge carriers in a device before any substantial non-geminate recombination has occurred. For devices that are still subject to geminate recombination, the measured values of L D represent the fraction of excitons which are able to be dissociated and extracted as photocurrent. Photovoltage thus provides a useful tool to probe exciton harvesting in dark excitonic materials which are inaccessible by conventional PL quenching techniques, while also offering insight into the recombination mechanisms responsible for non-unity charge collection efficiency. Device preparation Devices were fabricated on glass substrates, pre-patterned with a 150-nm-thick layer of indium-tin-oxide with a sheet resistance of 15 Ω per square. Each substrate was degreased by sonication in tergitol and acetone followed by boiling in isopropyl alcohol. Before thin film deposition, substrates were exposed to an ultraviolet-ozone atmosphere for 10 min. All device layers were fabricated using vacuum thermal sublimation/evaporation at pressures below 10 −6 Torr. The organic layers were deposited at 0.2 nm s −1 , and the Al cathode was deposited at 0.3 nm s −1 . All materials were used as received. Materials were obtained from the following suppliers: H 2 Pc and MgPc from Sigma-Aldrich; CuPc from Acros Organics; lead phthalocyanine from TCI America; BCP and Al from Alfa Aesar; SubPc from Luminescence Technology Corporation; and C 60 from MER Corporation. All devices were capped with a 10-nm-thick exciton blocking layer of BCP and a 100-nm-thick cathode layer of Al. All devices have an active area of 0.25 cm 2 . Charge extraction Charge extraction experiments were performed in atmosphere using an M455F1, M530F1, M625F1 or M735L3 LED from Thorlabs as the light source. The n-channel MOSFETs used to switch the LED and the OPV were manufactured by STmicroelectronics (STP27N3LH5). Integrated gate driver circuits were used to simultaneously switch the LED transistor and the OPV transistor. Since the transistors controlling the LED and the OPV must switch states in opposite directions at the same time, an inverting gate driver (Microchip Technology TC4421AVPA) was connected to the LED transistor and a non-inverting gate driver (Microchip Technology TC4422AVPA) was connected to the OPV transistor. The gate drivers were operated by the same pulses from an Agilent 33220A pulse generator, and the current transients were recorded using a Tektronix TDS5104B oscilloscope. Voltage transients Voltage transients were measured in atmosphere. The same LEDs used in the charge extraction experiment were used to obtain the voltage transients. The LEDs were powered by a Hewlett-Packard 8114A pulse generator, and the voltage transients were recorded by a Tektronix TDS5104B oscilloscope. The spectrum of each LED was measured using an Ocean Optics HR4000 spectrometer and the power output of the LEDs was recorded using a Thorlabs PDA36A amplified silicon photodetector. The values of L D obtained were (11.5±1.2) nm for C 60 , (8.5±1.0) nm for SubPc, (4.7±0.7) nm for H 2 Pc, (2.8±0.4) nm for MgPc, (4.7±0.7) nm for CuPc, and (4.6±0.9) nm for PbPc. Values of L D for a single device were determined by averaging three to five voltage transient measurements using LED intensities ranging from about 10 to 150 mW cm −2 . Reported L D values are obtained by averaging measurements of twelve C 60 , twelve SubPc, six H 2 Pc, three MgPc, fourteen CuPc and three PbPc devices. The error is the standard deviation across all devices and LED intensities. Computational notes The electric field in the device (used to extract L D from photovoltage measurements and to fit η EQE ) was calculated using a transfer matrix formalism previously described [20] . The layer thicknesses and optical constants needed as inputs to the model were measured using spectroscopic ellipsometry. The boundary conditions used to solve the exciton diffusion equation were a reflecting indium-tin-oxide–donor interface and an exciton sink at the donor-acceptor interface consistent with PL quenching-based measurements of L D . Data availability Data from this work is available from the corresponding author upon request. How to cite this article: Mullenbach, T. K. et al . Probing dark exciton diffusion using photovoltage. Nat. Commun. 8, 14215 doi: 10.1038/ncomms14215 (2017). Publisher's note: Springer Nature remains neutral with regard to jurisdictional claims in published maps and institutional affiliations.